Search for22Na in novae supported by a novel method for measuring femtosecond nuclear lifetimes Classical novae are thermonuclear explosions in stellar binary systems, and important sources of 26 Al and 22 Na. While γ rays from the decay of the former radioisotope have been observed throughout the Galaxy, 22 Na remains untraceable. Its half-life (2.6 yr) would allow the observation of its 1.275 MeV γ -ray line from a cosmic source. However, the prediction of such an observation requires good knowledge of its nucleosynthesis. The 22 Na( p , γ ) 23 Mg reaction remains the only source of large uncertainty about the amount of 22 Na ejected. Its rate is dominated by a single resonance on the short-lived state at 7785.0(7) keV in 23 Mg. Here, we propose a combined analysis of particle-particle correlations and velocity-difference profiles to measure femtosecond nuclear lifetimes. The application of this method to the study of the 23 Mg states, places strong limits on the amount of 22 Na produced in novae and constrains its detectability with future space-borne observatories. Nuclear reactions between charged particles in astrophysical environments proceed by quantum tunneling. The measurement of these reactions in the laboratory is very difficult because of the very small cross sections ( σ ≲ 1 nb). To date, about 10 reactions involving radioactive nuclei and charged particles have been directly measured at low energies. Among them, the 22 Na( p , γ ) 23 Mg reaction has a direct impact on the amount of radioactive 22 Na produced in novae [1] , [2] , [3] , [4] , [5] . The astrophysical relevance of 22 Na for the diagnosis of nova outbursts was first mentioned by Clayton and Hoyle [6] , in the context of its decay into a short-lived excited state of 22 Ne, and the subsequent emission of a γ -ray photon of 1.275 MeV released during its de-excitation. With the half-life of 22 Na being much longer than the transition time from an optically thick to an optically thin ejecta of a classical nova (about one week), the flux of the 1.275 MeV γ -ray line will remain close to its maximum value for months after the ejecta has become transparent to γ rays [7] . A precise determination of the 22 Na( p , γ ) 23 Mg thermonuclear rate is necessary to improve the predicted abundances of nuclei in the mass region A ≥ 20 during nova outbursts, including the 22 Na abundance in the ejecta that impacts in turn the predicted 20 Ne/ 22 Ne ratios in presolar grains [8] of a putative nova origin, as well as, the corresponding γ -ray emission flux. The rate of this reaction is mainly dictated by a single resonance in 23 Mg at 7785.0(7) keV [5] . A direct measurement of its strength ( ω γ ) has been performed in three different studies with conflicting results: \(\omega \gamma=5. {7}_{-0.9}^{+1.6}\) [5] , 1.8(7) [9] and <0.36 meV [10] . Indirect experimental methods, such as lifetime measurements, have also been employed to determine the strength of this resonance. Our simulations [11] show that, in the range of the debated values of the resonance strength, the mass of 22 Na ejected in novae depends on the lifetime ( τ ) of this key state approximately as M ejec ∝ τ 0.7 . The lifetime of this state was previously measured to be τ = 10(3) fs [4] , consistent with the recently determined upper limit of 12 fs [12] . Yet, this is at odds with the predictions of the nuclear Shell Model (SM), τ SM ≈ 1 fs. Here we propose an experimental method for measuring short ≈fs lifetimes. This method has been applied to the key state in 23 Mg in order to obtain an independent measurement and, so, to reduce systematic uncertainties. As a result, the rate of the 22 Na( p , γ ) 23 Mg reaction is now well known, and realistic estimates of the maximum detectability distance of novae in 1.275 MeV γ rays are derived. The experiment was performed at GANIL, France. A 24 Mg beam was accelerated to 110.8(4) MeV and impinged on a 3 He target of ≈2 × 10 17 atoms cm −2 uniformly implanted up to a depth of 0.1 μm below the surface of a 5.0(5) μm gold foil, producing the 23 Mg nucleus by the 3 He( 24 Mg, 4 He) 23 Mg reaction. Both 24 Mg and 23 Mg nuclei were then stopped in a 20.0(5) μm gold foil. The two gold foils were mounted back-to-back. About 20 states were populated in 23 Mg with excitation energies between 0 and 8 MeV. The light particles produced by the reaction were identified and measured with the VAMOS ++ magnetic spectrometer [13] placed at 0° with respect to the beam direction, using two drift chambers, a plastic scintillator and two small drift chambers placed at the entrance of the spectrometer. This led to an unambiguous identification of the 4 He particles. The 4 He particles were detected up to an angle in the laboratory of 10.0(5)° relative to the beam axis. The excitation energy ( E x ), the velocity at the time of the reaction ( β reac = v reac / c ), and the angle of the 23 Mg nuclei ( θ recoil ) have been determined by measuring the momentum of the 4 He ejectiles, with a resolution (FWHM) of ≈500 keV, ≈0.0005 and ≈ 0.05°, respectively. The excited states in 23 Mg have been also clearly identified via their γ -ray transitions measured with the \(\texttt{AGATA}\) γ -ray spectrometer [14] , [15] . The present experimental method has taken advantage of the highest angle sensitivity of \(\texttt{AGATA}\) [14] , [15] , shown in Fig. 1 b. This γ -ray spectrometer is based on γ -ray tracking techniques in highly segmented HPGe detectors. It consisted of 31 crystals covering an angular range from 120° to 170°, with a total geometrical efficiency ≈ 0.6 π . With \(\texttt{AGATA}\) , it is possible to measure accurately the energy and the emission angle of the γ rays with a resolution of 4.4(1) keV at 7 MeV and 0.7(1)°, respectively. The γ rays were observed Doppler shifted since they were emitted from a 23 Mg nucleus moving at a certain velocity β ems = v ems / c . The measured energy E γ is a function of β ems , of the center-of-mass energy E γ ,0 of the γ ray and of the angle θ between the γ ray and the 23 Mg emitting nucleus: \({E}_{\gamma }={E}_{\gamma,0}\sqrt{1-{\beta }_{{{{{{{{\rm{ems}}}}}}}}}^{2}}/(1-{\beta }_{{{{{{{{\rm{ems}}}}}}}}}\cos (\theta ))\) . With \(\texttt{AGATA}\) , this relativistic Doppler effect can be observed continuously as a function of the angle, as shown in Fig. 1 a for the case of the \({E}_{\gamma,0}=4840. {0}_{-0.4}^{+0.2}\) keV (we use energy values from the present measurement throughout this article) γ -ray transition emitted from the E x = 5292.0(6) keV excited state in 23 Mg moving with β ems ≈ 0.075. Conversely, if the center-of-mass energy of the γ ray is known, it is possible to determine the nucleus velocity at the time of emission β ems from the measured E γ and θ (see the “Methods” subsection “Determination of velocities”). Their precise measurement, enabled by the combination of both \(\texttt{AGATA}\) and \(\texttt{VAMOS}\) ++, has allowed for the accurate determination of β ems , on an event-by-event basis. Fig. 1: Identification of γ -ray transitions in 23 Mg. a The energy of the measured γ rays is plotted as a function of the angle between the γ ray and the 23 Mg emitter. This matrix is conditioned with the detection of an α particle at 5.2 < E x < 5.4 MeV in the VAMOS ++ magnetic spectrometer. The γ -ray transition ( \({E}_{\gamma,0}=4840. {0}_{-0.4}^{+0.2}\) keV) from the E x = 5292.0(6) keV excited state in 23 Mg is clearly observed. Its energy is Doppler shifted. The background observed here is mostly due to random coincidences between γ rays from the Compton background and α particles produced in fusion-evaporation reactions between the beam and 12 C and 16 O impurities deposited on the target. b Picture of the \(\texttt{AGATA}\) γ -ray spectrometer used to detect the γ rays emitted during the reaction. Full size image In the present work, both velocities β ems and β reac were measured simultaneously, on an event-by-event basis. The two velocities are not identical since (i) the 23 Mg nucleus slows down in the target before being stopped (≈500 fs) and (ii) there is a time difference between the reaction and the γ -ray emission due to the finite lifetime of the state. Thus, the profile of the velocity differences, Δ β = β reac − β ems , is a function of the lifetime of the state—a longer lifetime gives a larger value of Δ β . The technique proposed here, for measuring femtosecond lifetimes, is based on the analysis of velocity-difference profiles. The results obtained in this work are shown in Fig. 2 for three different excited states of 23 Mg. These measurements were made using an average beam intensity of 2 × 10 7 pps for a duration of ~132 h. In Fig. 2 a, β reac is shown as a function of β ems , and in (b), the yields of the corresponding γ rays as a function of the velocity difference Δ β . The overall shape of the Δ β measured profiles can be explained in a simple way. The γ rays are emitted following the exponential decay law, i.e. N ( t ) = N 0 × e −Δ t / τ , with τ being the lifetime of the state and Δ t the time elapsed after the reaction. For short lifetimes ( τ ≲ 100 fs), the deceleration acting on the 23 Mg ions is almost constant (d E /d x ≈ constant) and consequently Δ β ∝ Δ t . Therefore, the right side tail of the curves in Fig. 2 b would follow the exponential decay function N ( t ) ∝ e −Δ β / τ . This explains the asymmetric shape of the profile shown in blue, which corresponds to τ = 40 fs. Moreover, the experiment has a resolution in Δ β , i.e. 0.0032(1), which is measured by the width of the almost Gaussian profile observed for very short lifetimes, see the green profile for τ = 4 fs in Fig. 2 b. The overall shape of the measured Δ β distributions is the convolution of the exponential decay with a Gaussian function. The sensitivity of the method, governed by the statistics, can be better than the resolution of Δ β . This makes the method sensitive to very short lifetimes, down to 0.8 fs according to simulations. From comparison of the data with Monte Carlo simulations, shown in Fig. 2 b by the continuous lines (see also the Supplementary information ), the best agreement is obtained with lifetimes of \({4}_{-3}^{+1}\) and \(4{0}_{-7}^{+6}\) fs for the states E x = 5292.0(6) keV ( \({E}_{\gamma,0}=4840. {0}_{-0.4}^{+0.2}\) keV) and E x = 3796.8(12) keV ( \({E}_{\gamma,0}=3344. {8}_{-1.0}^{+0.8}\) keV), respectively, which is in excellent agreement with their known values of 5(2) [16] and 41(6) fs [16] . This shows that the present method is a powerful tool to determine lifetimes in the femtosecond range. With the same method, it is also possible to accurately measure the center-of-mass energy of the γ -ray transitions. For the transition from the key state ( E x = 7785.0(7) keV), we measured \({E}_{\gamma,0}=7333. {0}_{-0.2}^{+0.5}\) keV, in good agreement with the referenced value of E γ ,0 = 7333.2(11) keV [16] . Fig. 2: Angle-integrated velocity-difference profiles. a The 23 Mg velocity at the time of reaction ( β reac ) is shown against the velocity at the time of the γ -ray emission ( β ems ), for three excited states. The line corresponds to the prompt γ -ray emission when β ems = β reac . The points observed on the left of the line ( β ems < β reac ) correspond to delayed γ -ray emissions. b The corresponding angle-integrated velocity-difference profiles for the three states compared with simulations (continuous lines). It shows unambiguously that the key state (in red) has a lifetime 4 < τ < 40 fs. The red-shaded area corresponds to the simulations with lifetimes within 1 σ uncertainty. The horizontal error bars correspond to the width of the bins, which are larger than the real experimental uncertainty, and the vertical error bars to the statistical uncertainty. Full size image The present method has many advantages. Since the excitation energy of the state is selected with \(\texttt{VAMOS}\) ++, we can ignore any possible top-feeding contribution to the state, and, therefore, the measure is not affected by the lifetime of higher-lying states. Moreover, this method is independent of the reaction mechanism populating the states, i.e. direct transfer or compound-nucleus formation ( 24 Mg + 3 He → 27 Si * → 23 Mg + 4 He). Furthermore, the result does not depend on the angular distribution of the emitted γ ray and of the charged particles, nor on the angle-dependent detection efficiency. A single spectrum concentrates all the statistics of the experiment, which maximizes the signal-to-noise ratio. The statistical uncertainty on the lifetime of the key state is ~50%. 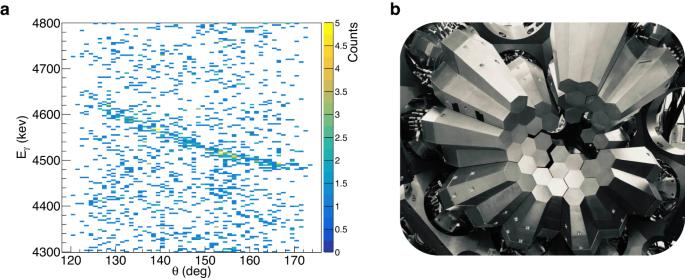Fig. 1: Identification ofγ-ray transitions in23Mg. aThe energy of the measuredγrays is plotted as a function of the angle between theγray and the23Mg emitter. This matrix is conditioned with the detection of anαparticle at 5.2 <Ex< 5.4 MeV in theVAMOS++ magnetic spectrometer. Theγ-ray transition (\({E}_{\gamma,0}=4840.{0}_{-0.4}^{+0.2}\)keV) from theEx= 5292.0(6) keV excited state in23Mg is clearly observed. Its energy is Doppler shifted. The background observed here is mostly due to random coincidences betweenγrays from the Compton background andαparticles produced in fusion-evaporation reactions between the beam and12C and16O impurities deposited on the target.bPicture of the\(\texttt{AGATA}\)γ-ray spectrometer used to detect theγrays emitted during the reaction. The main sources of systematic uncertainties are estimated to be 26% and the individual contributions are presented in Table 1 . Table 1 Systematic uncertainties (in %) on the lifetime of the key state Full size table The result obtained for the lifetime of the astrophysical state is \(\tau=1{1}_{-5}^{+7}\) fs, including statistical and systematic uncertainties (see Fig. 2 ), confirming the measured value of Jenkins et al. [4] ( τ = 10(3) fs). The reduced magnetic dipole transition probability B ( M 1) was deduced from the measured lifetime assuming a negligible E 2 electric quadrupole contribution: \(B(M1)=0.01{7}_{-0.008}^{+0.011}\,{\mu }_{N}^{2}\) . This value is among the lowest values measured for M 1 transitions. To get insight from theory, we have performed shell-model calculations in the s d shell with the well-established phenomenological USDA and USDB [17] , [18] interactions using the \(\texttt{NushellX@MSU}\) code [19] . These calculations confirm that the key state is characterized by a low B ( M 1) value of 0.14 \({\mu }_{N}^{2}\) , assuming 7/2 + spin and parity assignment (see the discussion below) and optimum values of the effective proton and neutron g -factors. Although this value is almost a factor of 10 larger than the experimentally determined one, the difference is not far from the typical rms error on M 1 transition probabilities established for the s d shell with these interactions [11] , [20] . Therefore, the measured values of the lifetime are compatible with shell-model calculations. The measured lifetime was used to determine the strength of the resonance: \(\omega \gamma=\frac{2{J}_{{}^{23}{{{{{{{\rm{Mg}}}}}}}}}+1}{(2{J}_{{}^{22}{{{{{{{\rm{Na}}}}}}}}}+1)(2{J}_{{\rm {p}}}+1)}\times \frac{{\Gamma }_{\gamma }{\Gamma }_{{\rm {p}}}}{{\Gamma }_{\gamma }+{\Gamma }_{{\rm {p}}}}=\omega {\rm {B{R}}}_{{\rm {p}}}(1-{\rm {B{R}}}_{{\rm {p}}})\frac{\hslash }{\tau }\) , with J and Γ being the spin and the partial widths of the key state. Actually, the spin of this state has also been a subject of debate [4] , [21] , where three values have been proposed: \({J}_{{}^{23}{{{{{{{\rm{Mg}}}}}}}}}^{\pi }=3/{2}^{+}\) [21] , 5/2 + [21] or 7/2 + [4] . We assume it to be 7/2 + . This state is only 18(1.5) keV away from the known 5/2 + isobaric analog state of the 23 Al ground state. In the case of the 5/2 + assignment, the states would interfere, as predicted by the nuclear shell-model calculations [11] , and such mixing has not been observed [5] , [9] , [22] , [23] . Moreover, concerning the γ -ray decay pattern, shell-model calculations agree with a 7/2 + spin [11] . The proton branching ratio, BR p , was also measured in this work by detecting protons emitted from the 23 Mg unbound states with an annular silicon detector placed downstream of the target (see Supplementary information ). The obtained value, BR p = 0.68(17)%, is in excellent agreement with the latest published value, BR p = 0.65(8)% [23] . Combining all measured values into the new recommended values: BR p = 0.66(7)% and τ = 10.2(26) fs, results in a consolidated resonance strength of \(\omega \gamma=0.2{4}_{-0.04}^{+0.11}\) meV, which is compatible with the direct measurement [10] ( ω γ < 0.36 meV) but not with the other two direct measurements. It should be pointed out that these direct measurements using radioactive targets are not in agreement with each other, and also that the obtained value is very low, close to the sensitivity limit of these direct experiments. The new value of the resonance strength and a Monte-Carlo approach [24] were used to deduce a new rate for the 22 Na( p , γ ) 23 Mg reaction (see Fig. 4 and Table 1 in Supplementary information ). The reliably estimated experimental uncertainties of the present method allowed a more accurate determination of this rate. This new rate was found to be very reliable at maximum nova temperatures, with uncertainties reduced to 40% (10%) at T = 0.1 GK (0.5 GK) (see Supplementary information ). To quantitatively assess the impact of the new 22 Na( p , γ ) 23 Mg reaction rate obtained from this work on nova nucleosynthesis, a series of hydrodynamic simulations have been performed. Four physical magnitudes determine the strength of a nova outburst, and, in turn, the synthesis of 22 Na: the white dwarf mass M WD (or radius R WD ), its initial luminosity L WD,ini , the mass-accretion rate \(\dot{M}\) , and the metallicity of the accreted material. The influence of the white dwarf mass on the synthesis of 22 Na has been analyzed. Three different values for the white dwarf mass have been considered: 1.15 M ⊙ , 1.25 M ⊙ , and 1.35 M ⊙ . In these simulations, the star hosting the nova outbursts is assumed to be an ONe white dwarf, with initial luminosity, L WD,ini = 10 −2 L ⊙ , and accreting solar composition material [25] from the secondary star at a constant mass-accretion rate of \(\dot{M}\) = 2 × 10 −10 M ⊙ /yr. The accreted matter is assumed to mix with material from the outermost white dwarf layers [26] . For consistency and completeness, the nova outbursts on 1.15 M ⊙ white dwarfs have been computed with two different, one-dimensional stellar evolution codes: \(\texttt{MESA}\) [27] , [28] , [29] , [30] , [31] , [32] and \(\texttt{SHIVA}\) [33] , [34] . At the early stages of the outburst, when the temperature at the base of the envelope reaches T base ~ 5 × 10 7 K, the chain of reactions 20 Ne( p , γ ) 21 Na( β + ) 21 Ne( p , γ ) 22 Na powers a rapid rise in the 22 Na abundance. When the temperature reaches T base ~ 8 × 10 7 K, 22 Na( p , γ ) 23 Mg becomes the main destruction channel. At T base ~ 10 8 K, 22 Na( p , γ ) 23 Mg becomes the most important reaction involved in the synthesis and destruction of 22 Na, and therefore, its abundance begins to decrease. 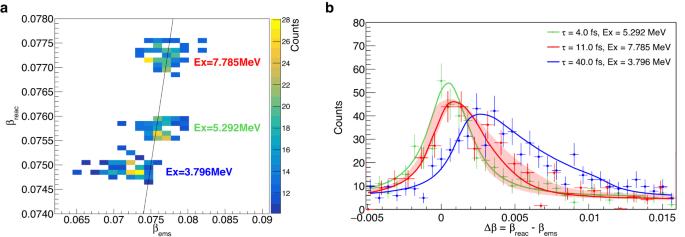Fig. 2: Angle-integrated velocity-difference profiles. aThe23Mg velocity at the time of reaction (βreac) is shown against the velocity at the time of theγ-ray emission (βems), for three excited states. The line corresponds to the promptγ-ray emission whenβems=βreac. The points observed on the left of the line (βems<βreac) correspond to delayedγ-ray emissions.bThe corresponding angle-integrated velocity-difference profiles for the three states compared with simulations (continuous lines). It shows unambiguously that the key state (in red) has a lifetime 4 <τ< 40 fs. The red-shaded area corresponds to the simulations with lifetimes within 1σuncertainty. The horizontal error bars correspond to the width of the bins, which are larger than the real experimental uncertainty, and the vertical error bars to the statistical uncertainty. 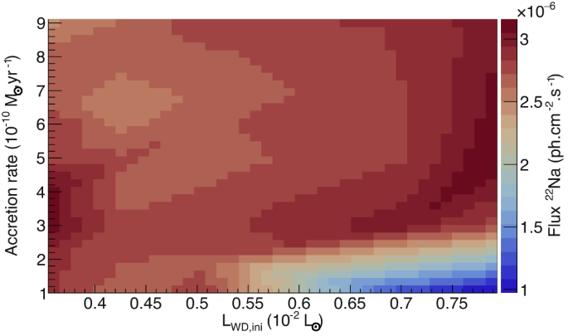Fig. 3: Prediction of the 1.275 MeVγ-ray flux emitted from a nova. The22Naγ-ray emission flux is shown as a function of the white dwarf initial luminosity and the mass-accretion rate. This is calculated from the22Na mass-averaged abundance within the ejected shells. Computations were done for a 1.2M⊙ONe white dwarf located 1 kpc from the Earth, using the\(\texttt{MESA}\)code27,28,29,30,31,32. When T base ~ 2 × 10 8 K, 21 Na( p , γ ) 22 Mg becomes faster than 21 Na( β + ) 21 Ne, such that 20 Ne( p , γ ) 21 Na( p , γ ) 22 Mg( β + ) 22 Na takes over as the dominant path, favoring the synthesis of 22 Na, which achieves a second maximum after the temperature peak T peak (see Table 2 ). This pattern continues up to 22 Na( p , γ ) 23 Mg becomes again the most relevant reaction when the temperature drops. During the subsequent and final expansion and ejection stages, as the temperature drops dramatically, the evolution of 22 Na is fully governed by 22 Na( β + ) 22 Ne. The most relevant results obtained in these simulations are summarized in Table 2 . The larger peak temperatures achieved during nova outbursts on more massive white dwarfs yield larger mean, mass-averaged abundances of 22 Na in the ejecta. However, it is worth noting that the total mass of 22 Na ejected in a nova outburst decreases with the white dwarf mass (8 × 10 −9 M ⊙ , for Model 115b, 7 × 10 −9 M ⊙ , for Model 125, and 4.2 × 10 −9 M ⊙ , for Model 135), since more massive white dwarfs accrete and eject smaller amounts of mass, see M ejec in Table 2 . Table 2 Abundances of (Ne, Na) isotopes in the ejecta obtained for different nova models calculated with the \(\texttt{MESA}\) and \(\texttt{SHIVA}\) codes (see text for the parameters) Full size table The new and reliable reaction rate obtained in this work also opens the door to further advanced sensitivity studies on astrophysical parameters, performed here for the first time. The flux has been obtained in a series of nova simulations for a large range of mass-accretion rates \(\dot{M}\) and white dwarf luminosities L WD,ini . For example, Fig. 3 shows the expected flux of 22 Na for a nova event located 1 kpc from the Earth, with M WD = 1.2 M ⊙ and accreting solar composition material. This figure shows that the amount of 22 Na does depend on the two parameters, varying smoothly by up to a factor of 3. The change is abrupt only on the lower right side of the figure. In this region, the 22 Na/ 22 Mg and 22 Na/ 21 Ne ratios around the peak temperatures have the same values as in the other regions, which means that the production pathways are unchanged. On the contrary, the 23 Mg/ 22 Na ratio is found 4 times larger, indicating that the destruction by the 22 Na( p , γ ) 23 Mg reaction is more intense in this region. This graph provides a link between the unknown astrophysical parameters of the novae and the predicted 22 Na flux. In the future, precise measurements of the 22 Na γ -ray flux will constrain these astrophysical parameters. Fig. 3: Prediction of the 1.275 MeV γ -ray flux emitted from a nova. The 22 Na γ -ray emission flux is shown as a function of the white dwarf initial luminosity and the mass-accretion rate. This is calculated from the 22 Na mass-averaged abundance within the ejected shells. Computations were done for a 1.2 M ⊙ ONe white dwarf located 1 kpc from the Earth, using the \(\texttt{MESA}\) code [27] , [28] , [29] , [30] , [31] , [32] . Full size image New instruments for γ -ray astronomy are under study or under construction: ESA’s enhanced e-ASTROGAM [35] and NASA’s COmpton Spectrometer and Imager, COSI [36] . Both are, in principle, capable of detecting the 1.275 MeV γ rays released in the decay of 22 Na produced in nova outbursts, since they are being designed with a higher efficiency than the past missions, INTEGRAL-SPI [37] and COMPTEL-CGRO [38] . The very high precision in the determination of the 22 Na( p , γ ) 23 Mg rate reported in this work permits deriving, for the first time, realistic estimates of the maximum detectability distance of novae in γ rays, through the 1.275 MeV line. With the expected sensitivities of e-ASTROGRAM (3 × 10 −6 photons cm −2 s −1 ) and COSI (1.7 × 10 −6 photons cm −2 s −1 ) at 1 MeV, and assuming model 125 (Table 2 ), the new maximum detectability distances of 2.7 and 4.0 kpc, respectively, have been derived, on which the reaction rate uncertainty obtained here leads to an uncertainty of 18%. These new estimates suggest a large chance for the possible detection of the 22 Na γ rays produced in ONe novae by the next generation of space-borne γ -ray observatories. Determination of velocities The velocity β reac of the 23 Mg nuclei at the reaction time was derived from the momentum of the α particles measured with the VAMOS ++ magnetic spectrometer and from the kinematics laws of energy and momentum conservation in the case of the 3 He( 24 Mg, α ) 23 Mg two-body reaction 
    β_reac=√(1-γ_reac^-2)
 (1) with 
    γ_reac=√(1+m_α^2β_α^2/1-β_α^2+m_beam^2β_beam^2/1-β_beam^2-2cos (θ_α)m_beamm_α√(γ_α^2-1)√(γ_beam^2-1)/m_recoil^2)
 (2) where m α , m beam and m recoil are the rest-mass energies of the α , 24 Mg, and 23 Mg nuclei, θ α the angle between the α particle and the beam axis. The parameter γ α was measured with VAMOS ++ and corrected for the energy losses in the target using the \(\texttt{SRIM}\) code [39] . The parameter γ beam was measured prior to the experiment, γ reac was then determined from the measured γ α and a γ -ray transition was detected in coincidence. The velocity β ems of the 23 Mg nuclei at the γ -ray emission time was derived from the measured γ rays. Since the 23 Mg nuclei are moving at the time of the γ -ray emission, the γ -ray energy is Doppler shifted, with the measured energies E γ shifted from the center-of-mass energy E γ ,0 according to 
    E_γ=E_γ,0√(1-β_ems^2)/1-β_emscos (θ )
 (3) It follows that 
    β_ems=R^2cos (θ )+√(1+R^2cos^2(θ )-R^2)/R^2cos^2(θ )+1
 (4) with R = E γ / E γ ,0 . Here, R < 1 since the \(\texttt{AGATA}\) detector was located upstream of the target. The angle θ between the γ ray and the 23 Mg recoil nucleus was derived from the measured ( θ , ϕ ) of the γ ray and the α particle using the formulas 
    cos (θ )=	sin (θ_γ)sin (θ_recoil)[cos (ϕ_γ)cos (ϕ_recoil) 
     	+sin (ϕ_γ)sin (ϕ_recoil)]+cos (θ_γ)cos (θ_recoil)
 where 
    θ_recoil=acos(m_beam√(γ_beam^2-1)-m_αcos (θ_α)√(γ_α^2-1)/m_recoil√(γ_recoil^2-1))  and ϕ_recoil=π+ϕ_α
 Fit of velocity-difference profiles Velocity-difference profiles were numerically simulated with a Monte-Carlo approach developed in the \(\texttt{EVASIONS}\) C++/ROOT code [40] . Simulated velocity-difference profiles were normalized to the measured ones via the profile integrals. The goodness of fit between experimental and simulated profiles was quantified with the Pearson χ 2 tests where the lifetime and the γ -ray center-of-mass energy were taken as free parameters. Branching ratios The E x = 7785.0(7) keV astrophysical state can decay via proton or γ -ray emission. Therefore, after applying a selection on E x in 23 Mg by using the measured α particles, the number of detected protons and γ rays allowed us to determine the proton and γ -ray branching ratios. These values were corrected for detection efficiencies. On the one hand, the geometrical efficiency of the silicon detector was estimated by numerical simulations. The angular distribution was considered isotropic for the emitted ℓ = 0 protons. On the other hand, the \(\texttt{AGATA}\) efficiency was measured at low energies with a radioactive 152 Eu source, and simulated with the \(\texttt{AGATA}\) \(\texttt{Geant4}\) code library [41] , [42] to determine the efficiency at high energies after scaling the simulations to the measured efficiencies at low energies. Determination of the 22 Na flux in novae The amount of 22 Na ejected in a nova outburst was obtained with the simulation codes \(\texttt{MESA}\) [27] , [28] , [29] , [30] , [31] and \(\texttt{SHIVA}\) [33] , [34] from its abundance in the ejected layers. \(\texttt{SHIVA}\) and \(\texttt{MESA}\) use two basic criteria for the ejection of a specific layer: if its velocity achieves the escape velocity (~1000 km s −1 ), or if its luminosity becomes higher than the Eddington limit (when the force exerted by radiation exceeds the gravitational pull) and hence, the condition of hydrostatic equilibrium no longer holds.